Two-photon polarization-selective etching of emergent nano-structures on diamond surfaces Optical techniques have advanced considerably in recent years to enable processing of surfaces with a resolution less than the wavelength of light. Despite the highly selective nature of light-matter interactions, however, efforts to increase resolution to the scale of single atoms are hampered by rapid and efficient dissipation of the absorbed energy to the surrounding matrix. Here we show that two-photon surface excitation using ultraviolet light provides a method for selectively removing carbon from diamond surfaces. Polished surfaces etched by this method develop ultra-deep subwavelength structures with morphologies dependent on the polarization of the incident laser with respect to the crystal axes. As well as revealing a practical and versatile method for nano-patterning of diamond surfaces, we show that the results comprise mesoscopic evidence for bond scission via a highly localized optical interaction that may lead to the development of new optical approaches for ultra-nanoscale (<10 nm) surface structuring. Manipulation of single or groups of atoms on surfaces has enormous potential for the development of future nano-scale devices. Currently, the most powerful examples of atom-scale manipulation involve the use of forces and currents at the apex of sharp tips in scanning probe microscopy [1] , [2] . However, these techniques are often unsuited to the strongly bound and electrically insulating nature of many covalently bonded materials. In contrast, strong covalent bonds offer the advantage that the associated bonding electrons comprise highly localized oscillators that can be targeted resonantly using light. Single bonds between carbon atoms, for example, carry electronic absorption signatures that are relatively unperturbed by the neighbouring bonding environment [3] , [4] . Therefore, light, with all its practical conveniences, has the potential to extend resolution below the subwavelength scales already seen [5] , [6] , [7] and to enable targeted bond breakage and atom manipulation for materials incompatible with current scanning probe methods. To date, only bonds in gas phase species or between H adsorbates on Si surfaces have exhibited photo-selective bond scission [8] , [9] , [10] . We have investigated single-crystal diamond as a promising candidate for revealing photo-selective scission of structural bonds in a strong covalently bound system. In this respect, diamond is ideal. It presents a simple symmetrical structure of sp3 -bonded carbon atoms while being also a material of enormous interest in science and technology [11] , [12] , [13] , [14] , [15] , [16] , [17] . Furthermore, diamond exhibits an unusual mode of carbon removal from the surface when excited by photons of energy approaching the bandgap. It has been shown that carbon atoms are ejected from the surface when using wavelengths near 250 nm (refs 18 , 19 ) at a rate consistent with a two-photon excitation mechanism [18] and a cross-section of approximately 20 Goeppert-Mayers. The two-photon dependence, along with a lack of threshold, is indicative of a material ejection mechanism intrinsically different from usual laser ablation and desorption which rely upon thermal- or plasma-mediated ejection mechanisms. The process is also distinguished from laser ablation of diamond by the absence of graphite formation on the treated surface [18] , [19] . Here we show that the two-photon-induced ejection mechanism in diamond involves light coupling with localized states that preserve the light polarization information. We find that the ejection probability displays a strong dependence on the light polarization with respect to the lattice bond directions. By repetitive pulsed exposure of the surface, these properties are revealed as deep-subwavelength patterns etched into the surface that exhibit striking variations in morphology as the polarization is rotated with respect to crystal axes. Patterning of {100} and {110} surfaces Diamond single crystals were exposed to 266 nm laser pulses at fluences approximately half of the ablation threshold. By etching to depths of several hundred nanometers, patterns were clearly resolved by electron microscopy. For a diamond cubic face with light at normal incidence, the nano-pattern polarization dependence can be effectively characterized by considering three crystal directions of high symmetry as shown in Fig. 1 . When the polarization is parallel to [110] ( E ||[110]), the pattern consists of faceted ridges oriented perpendicular to the polarization ( Fig. 1b ). The ridges are quasi-regular with a spatial frequency in the range 0.3–4 λ p −1 , where λ p =266 nm is the laser wavelength. More complex patterns are obtained when using polarization away from the [110] direction. For E ||[210] ( Fig. 1c ), the average ridge direction is approximately 4.5 degrees from the [110] direction and no longer perpendicular to the laser polarization. The ridges are narrower, exhibit more bifurcations and contain spatial frequencies extending up to 5 λ p −1 . When aligned along the cubic direction E ||[100] ( Fig. 1d ), the pattern consists of a cross hatched or grid-like structure oriented within a few degrees of [110]. Spatial frequencies up to 4–5 λ p −1 appear in the vertical and horizontal directions. Feature sizes as short as 50 nm are clearly observed in the magnified inset image. The contrast in the spatial frequency content for each image is clearly visible in the two-dimensional power spectra shown in Fig. 2 . Upon rotation of the writing beam polarization by angles beyond [100], the pattern reverts progressively to resemble again those identified for E ||[210] and [110], except reflected about the [100] axis in accordance with the C 4 rotational symmetry of the lattice surface. 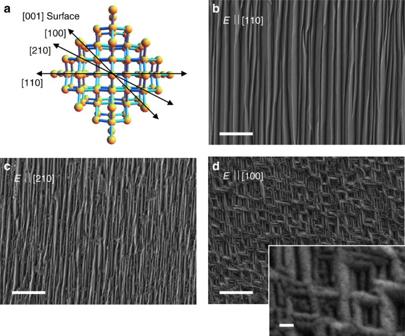Figure 1: Patterning of the {001} surface. (a) Polarization and lattice bond directions as viewed in the direction of the incident laser beam. (b–d) 6.0 × 4.5 μm Images for a laser beam at normal incidence with polarizations parallel to [110], [210] and [100]. Scale bars, 1,000 nm, except for inset of (d), 100 nm. In each case the laser dose was 10.3 MJ cm−2, and the average depth of material removed was 550 nm. The inset image contains a close-up view (0.97 × 0.65 μm) of the pattern ind. Figure 1: Patterning of the {001} surface. ( a ) Polarization and lattice bond directions as viewed in the direction of the incident laser beam. ( b – d ) 6.0 × 4.5 μm Images for a laser beam at normal incidence with polarizations parallel to [110], [210] and [100]. Scale bars, 1,000 nm, except for inset of ( d ), 100 nm. In each case the laser dose was 10.3 MJ cm −2 , and the average depth of material removed was 550 nm. The inset image contains a close-up view (0.97 × 0.65 μm) of the pattern in d . 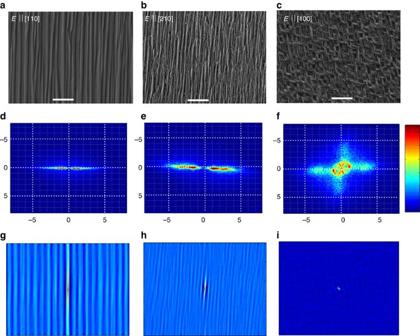Figure 2: Pattern spatial frequency and long range order for the (001) surface. The raw images (a–c) are reproduced in the top-row for ease of comparison. Corresponding power spectra (d–f) and auto-correlations (g–i) for the (001) surface images ofFig. 1. Frequencies are expressed in reciprocal laser wavelengths. Scale bars, 1 μm. Full size image Figure 2: Pattern spatial frequency and long range order for the (001) surface. The raw images ( a – c ) are reproduced in the top-row for ease of comparison. Corresponding power spectra ( d – f ) and auto-correlations ( g – i ) for the (001) surface images of Fig. 1 . Frequencies are expressed in reciprocal laser wavelengths. Scale bars, 1 μm. Full size image The contrasting symmetry and distribution of local environments for atoms on a {110} surface are also evident in the etched patterns. Three pattern types distinct from those for the {100} face were obtained for polarizations parallel to the low Miller index directions [001], [111] and [110] ( Fig. 3 ). For E ||[001], faceted ridges of spatial frequency approximately 1.6 λ p −1 were formed with direction perpendicular to the polarization. In contrast to the ridges observed on the {100} face, these faceted ridges exhibit stepped dislocations along each ridge spaced by about 1 μm. For E ||[111], parallel running ridges are also observed but have a complex unfaceted cross-sectional shape and a direction approximately 45° from [001] and 80° from the laser polarization direction. The pattern for E||[110] consists of a ripple pattern of similar spatial frequency ( Fig. 4 ), but in this case the ripples are more sinusoidal and once again aligned perpendicular to the laser polarization. 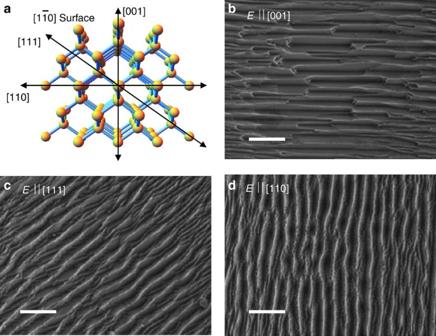Figure 3: Patterning of the {110} surface. (a) Polarization and lattice bond directions as viewed in the direction of the incident laser beam. (b–d) 3.0 × 2.25 μm images for laser polarizations parallel to [001], [111] and [110] directions. Scale bars, 500 nm. The laser dose was 10.8 MJ cm−2in each case. The etch depths were 350 nm, 510 nm and 530 nm, respectively. Figure 3: Patterning of the {110} surface. ( a ) Polarization and lattice bond directions as viewed in the direction of the incident laser beam. ( b – d ) 3.0 × 2.25 μm images for laser polarizations parallel to [001], [111] and [110] directions. Scale bars, 500 nm. The laser dose was 10.8 MJ cm −2 in each case. The etch depths were 350 nm, 510 nm and 530 nm, respectively. 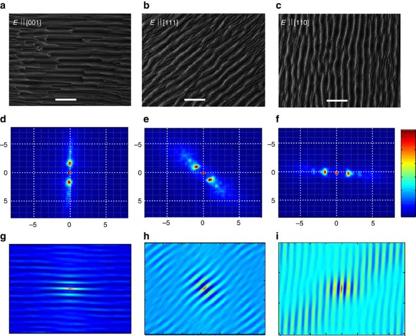Figure 4: Pattern spatial frequency and long range order for the (110) surface. The raw images (a–c) are reproduced in the top-row for ease of comparison. Corresponding power spectra (d–f) and auto-correlations (g–i) for the surface images ofFig. 3. Frequencies are expressed in reciprocal laser wavelengths. Scale bars, 500 nm. Full size image Figure 4: Pattern spatial frequency and long range order for the (110) surface. The raw images ( a – c ) are reproduced in the top-row for ease of comparison. Corresponding power spectra ( d – f ) and auto-correlations ( g – i ) for the surface images of Fig. 3 . Frequencies are expressed in reciprocal laser wavelengths. Scale bars, 500 nm. Full size image The patterns of Figs 1 and 3 are representative of the polarization dependence observed for the hundreds of etches we carried out on several diamond substrates with nitrogen content in the range 20–100 p.p.b. Polarizations along 〈1 yz 〉 crystal directions where y , z =0 or 1 produce the simplest patterns–that is, those easily identifiable as ridges, ripples or grids. These patterns often exhibit good long-range order (See Figs 2g–i and 4g–i ). We noted that facetted ridges are generally obtained when the laser polarization is parallel to projections of 〈111〉 on the surface plane. Scanning probe microscopy indicates that the facet angles are often consistent with {111} and {221} surfaces as shown, for example, for a {100} surface etched with E ||〈110〉 ( Fig. 5 ). 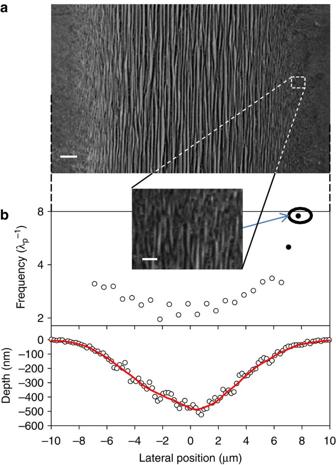Figure 5: Pattern formation across a photo-etched trench on a (100) surface. (a) 17.2 × 12.9 μm SEM image of a trench etched for E||〈110〉 showing the decrease in spatial frequency with etch depth. The trench was created using a rastered beam in the vertical direction 30 passes spaced by 2 μm. Periodic structures spaced by 20 nm are observed at the trench fringe as shown in the inset image. Scale bar, 1,000 nm, inset image, 100 nm. (b) Frequency expectation value of the 1-D power spectrum as a function of lateral position (top) and etch depth (bottom). For positions more than 6.5 μm from the trench axis, frequencies were obtained using higher magnification images (solid symbols). Figure 5: Pattern formation across a photo-etched trench on a (100) surface. ( a ) 17.2 × 12.9 μm SEM image of a trench etched for E||〈110〉 showing the decrease in spatial frequency with etch depth. The trench was created using a rastered beam in the vertical direction 30 passes spaced by 2 μm. Periodic structures spaced by 20 nm are observed at the trench fringe as shown in the inset image. Scale bar, 1,000 nm, inset image, 100 nm. ( b ) Frequency expectation value of the 1-D power spectrum as a function of lateral position (top) and etch depth (bottom). For positions more than 6.5 μm from the trench axis, frequencies were obtained using higher magnification images (solid symbols). Full size image Factors influencing morphology and frequency Pattern development is a function of depth and depends only weakly on laser fluence in the investigated range of 2–50 J cm −2 . For small etch depths, the patterns exhibit random structure of high spatial frequency, that progress to clear regular structures of lower frequency with further removal of material ( Fig. 6 ). With the field emission electron microscope, we were able to resolve feature sizes as small as 10–20 nm as shown in the inset image of Fig. 6a . The increase in spatial frequency at the fringes of the pattern suggests that much smaller features are created for very small etch depths. Pattern evolution was observed to proceed in the same way across all parts of the beam cross-section. We rule out beam back reflection from the second surface of the sample as a major influence on pattern development; the observed decrease in pattern spatial frequency on etch depth is inconsistent with an interferometric mechanism. Furthermore, identical patterns were reproduced on sample thicknesses from 1.5 to 22 Rayleigh ranges, for which the retro-reflected intensities of the incident beam decrease from 5.5 to 0.03%. No change in pattern was visible when varying angle of incidence by up to 5°. 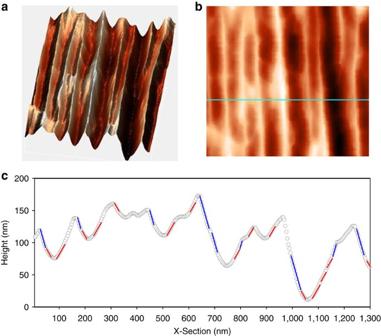Figure 6: Faceting on the {100} surface. (a) 3-D and (b) 2-D AFM images of a 1.3 × 1.3 μm area in an etched pattern with E||110] (as inFig. 1b). (c) The image cross-section for the horizontal line shown in (b). The solid lines indicate portions of the cross-section that fall closely within {111} (blue) and {221} (red) planes. Figure 6: Faceting on the {100} surface. ( a ) 3-D and ( b ) 2-D AFM images of a 1.3 × 1.3 μm area in an etched pattern with E||110] (as in Fig. 1b ). ( c ) The image cross-section for the horizontal line shown in ( b ). The solid lines indicate portions of the cross-section that fall closely within {111} (blue) and {221} (red) planes. Full size image The observed patterning has starkly contrasting properties to the laser-induced periodic surface structuring observed, to date, in any material [20] , [21] , [22] , [23] , [24] , [25] , [26] , [27] including diamond [20] , [28] , [29] , [30] , [31] . For incident intensities near the ablation threshold or at the fringes of an ablation spot, ripple-like structures are produced with periodicity approximately equal to the wavelength of the incident light and with direction perpendicular to the laser polarization, except in a few special cases that combine angle of incidence and polarization to perturb the pattern symmetry [25] , [27] . For studies on single-crystal substrates [20] , [21] , [27] , [28] , [29] , [30] , no lattice-polarization angle dependence was observed. To date, ripple formation has been explained in terms of interference effects between the light beam and the light-induced waves established on the heated surface [32] , [33] . In our case, the pattern morphologies are much more diverse according to the crystal orientation and much higher spatial frequencies are obtained. The influence of crystal orientation is most evident on the cubic face where the periodic structures show a closer relationship with the bond directions ( Fig. 1b–d ) than to the laser polarization. For the special case of E ||[100], where the polarization has an equal projection along all bonds, the grid pattern is aligned to surface projections of carbon-carbon lattice bonds and the pattern shares the C 4 point symmetry of the surface ( Fig. 1d ). We found that the same grid structure and orientation were reproduced using circular polarization, which likewise projects an equal polarization along all lattice bonds. The pattern type and orientation is thus principally determined by the overlap between the polarization and directional surface states, rather than collective surface wave excitations of previous laser-induced patterns [20] , [21] , [22] , [23] , [24] , [25] , [26] , [27] , [28] , [29] , [30] , [31] , [32] , [33] . Our observations of structures with period less than 20 nm for small etch depths are consistent with a highly localized light-material interaction. We propose that the patterns develop as a result of anisotropic coupling of photons with surface bonds in convolution with a probability for carbon ejection dependent on the local bonding environment. As carbon removal progresses, the spatially dependent ejection probability becomes visible on the mesoscale in the form of patterns containing symmetries of the lattice surface. The rich variety of patterns produced as functions of facet and polarization reveal that the ejection probability is a complex function of the local surface structure and beam polarization. Such an ejection mechanism is consistent with the thresholdless and ‘cold’ nature of the process, and is distinct from the exponential and thermal nature of the periodic structuring observed previously [20] , [21] , [22] , [23] , [24] , [25] , [26] , [27] , [28] , [29] , [30] , [31] , [32] , [33] , [34] , [35] when using higher intensities, either near or above the ablation threshold. Further work is needed to determine whether bond scission results from direct coupling of the ultraviolet with carbon–carbon bonds or is reliant on cooperative processes with electronic states associated with surface reconstructions, radical sites or chemisorbed atoms. For example, the two-photon excitation may occur via gap-state resonances [34] associated with these surface configurations. The polarization-dependent ejection probability demonstrated here is a novel phenomenon with implications in photochemistry, surface physics and laser surface structuring. As the process can be performed in ambient conditions, it provides a straightforward and area-scalable method for tailoring the nano-scale morphology of diamond surfaces. This may be of direct interest in areas such as ultralow friction surfaces [15] , biochemical substrates [14] , and surface-enhanced ultrasensitive molecular sensors [35] . Of more fundamental importance, the evidence for coupling between the light field and localized bonds reveals promise for developing optical tools for bond-specific manipulation in covalent materials. Such manipulation on dimensions approaching the atomic scale may be made possible in future using, for example, tip-enhanced nano-optical techniques [36] , [37] . This may provide a pathway forward for engineering diamond devices that benefit from increased resolution such as low-loss waveguides [38] , quantum devices [11] , [12] , [13] , [39] , high-speed electronics [40] and high-density data storage [41] . Sample etching The single-crystal samples were Type IIa diamond of rms roughness 1 nm (Optical Grade, Element 6) and cleaned using a piranha chemical solution before UV exposure. The UV beam from a 266 nm laser of pulse duration 11 ns full-width-half maximum and repetition rate 13-14 kHz was focused to a waist radius of 4.8 μm on the sample top surface using a 25 mm focal length objective. The fluence was selected to be approximately 50% below the ablation threshold of 100 J cm −2 , which provided etch rates of approximately 10 nm per second without risk of ablation. The ablation threshold is defined here as the fluence at which there is a 50% probability for explosive material removal for a burst of 10 3 pulses. The two-photon cross-section of 20 GM was evaluated using the measured [18] etch rate of 3 pm per pulse from the {100} surface for a beam with a pulse fluence of 60 J cm −2 , spot-size 4.8 μm and pulse duration 11 ns. For this calculation, the carbon atom surface density was taken as twice the unit cell surface density. The sample was accurately positioned and rastered using a computer-controlled positioning stage. The polarization was aligned by rotation of the sample on the stage against facet orientation specified by the manufacturer and confirmed by us using polarized Raman spectroscopy. Surface analysis Etch depths were measured using an optical profiler (VEECO, Wyko NT3300, 514 nm, Objective NA=0.85). Pattern images were obtained using a field-emission SEM (JEOL JSM-7800 F). The SEM electron voltage was 2 kV, which we found provided the best resolution and minimal image distortion of the UV-treated diamond surface. Pattern profiles were obtained by atomic force microscopy (MT-NDT Ntegra Spectra) in non-contact mode using a Si tip of radius of curvature 10 nm (NT-MDT NSG01). Image analysis software (Image Analysis 3, NT-MDT) was used to reduce the effects of the finite tip radius. How to cite this article: Lehmann, A. et al. Two-photon polarization-selective etching of emergent nano-structures on diamond surfaces. Nat. Commun. 5:3341 doi: 10.1038/ncomms4341 (2014).